Selective cancer targeting with prodrugs activated by histone deacetylases and a tumour-associated protease Eradication of cancer cells while minimizing damage to healthy cells is a primary goal of cancer therapy. Highly selective drugs are urgently needed. Here we demonstrate a new prodrug strategy for selective cancer therapy that utilizes increased histone deacetylase (HDAC) and tumour-associated protease activities produced in malignant cancer cells. By coupling an acetylated lysine group to puromycin, a masked cytotoxic agent is created, which is serially activated by HDAC and an endogenous protease cathepsin L (CTSL) that remove the acetyl group first and then the unacetylated lysine group liberating puromycin. The agent selectively kills human cancer cell lines with high HDAC and CTSL activities. In vivo studies confirm tumour growth inhibition in prodrug-treated mice bearing human cancer xenografts. This cancer-selective cleavage of the masking group is a promising strategy for the next generation of anticancer drug development that could be applied to many other cytotoxic agents. A major challenge of current cancer therapies is to improve their selectivity against tumour cells. Most chemotherapeutic agents perturb functions that are common to both tumour and normal cells, resulting in limited therapeutic efficacy due to their adverse side effects. Therefore, drugs with improved selectivity are urgently needed to eliminate cancer cells, while leaving healthy cells unharmed. Histone deacetylases (HDACs) are key enzymes involved in the epigenetic modulation of histone and non-histone proteins [1] . HDACs modulate protein structure and function through deacetylation of lysine residues. In cancer biology, the involvement of HDACs has been well documented, supporting the notion that altered expression of HDACs could have an active role in tumour development [2] , [3] . Consistent with this, the therapeutic potential of HDAC inhibitors (HDACi) is recognized as a new class of drug for cancer [3] , [4] , [5] . Currently, a number of HDACi are in clinical trials for various haematologic and solid tumours [5] , [6] . However, certain HDACs are essential for normal cells and a therapeutic approach using these pharmacologic inhibitors depends on the tolerance levels of normal cells to the damage caused by the treatment [7] , [8] . Tumour-associated cysteine protease cathepsin L (CTSL) also has crucial roles at multiple stages of tumour progression and metastasis [9] , [10] , [11] . Cell lines transformed by certain oncogenes, including ras, are known to express high levels of CTSL [12] , [13] , [14] . Thus, the upregulation of CTSL is recognized as a hallmark of metastatic cancers and could be utilized as a prognostic marker [9] , [10] , [11] , [15] , [16] . Recently, nuclear-localized CTSL involved in cancer has been revealed, suggesting that CTSL may have key roles in the nucleus beyond its known lysosomal and extracellular activities [11] , [16] , [17] , [18] , [19] . Although the therapeutic potential of CTSL inhibitors has not been fully characterized in preclinical studies, targeting CTSL activity is considered as a strategy for anticancer therapy [20] . On the basis of the accumulating evidence [21] , [22] , [23] , certain tumour cells are more reliant on their elevated level of HDACs to survive and proliferate under stressful conditions. Thus, we explored taking advantage of the increased activities of HDACs and CTSL as a selective modality for delivering therapeutics to cancer cells instead of using inhibitors. Although many peptide-based prodrugs activated by tumour-associated proteases have been developed [24] , stability and nonspecific activation of parental drugs due to ubiquitous proteases are key factors limiting their clinical efficacy. By introducing an ε-acetylated lysine as the first requirement, the resulting prodrug is expected to be well-protected from proteolytic cleavage until it is deacetylated by the intracellular HDAC, and thus enables highly selective activation in tumour tissues. In this report, we describe a novel prodrug strategy targeting increased HDAC and CTSL activities in malignant tumours. In vitro proof-of-concept studies show that the prodrug exerts promising anticancer efficacy in a wide range of cancer cells. Further studies on mouse xenograft models bearing human colon cancer confirm the anticancer activity of the prodrug by its ability to inhibit tumour growth without severe adverse effects. The cancer-selective cleavage of the small-molecule masking group may serve as a promising strategy for next generation of anticancer drug development. Increased HDAC and CTSL activities in cancer cells To test whether increased activities of HDAC and CTSL provide a selective environment for targeted cancer therapy, we screened cancer cells for elevated levels of enzymes by measuring respective HDAC and CTSL activity in a panel of human cancer cell lines, including colon cancer (Caco-2, COGA-10 (ref. 25 ), HCA-7, HT29 and HCT116), pancreatic cancer (BXPC3 and MiaPaca-2), liver cancer HepG2 and cervical cancer HeLa, as well as non-tumorigenic human colon epithelial cells CCD841-CoN and normal mouse mammary epithelial cells Eph4 (ref. 26 ; Fig. 1a,b ). Using a standard HDAC assay, we observed marked high levels of HDAC activity in all malignant cell lines tested and, in clear contrast, low levels in less tumorigenic and normal cell lines (Caco-2, CCD841-CoN and Eph4; Fig. 1a ). The specificity of the HDAC assay was confirmed with inclusion of a HDACi Trichostatin A (TSA) [27] . Although Caco-2 cells originate from human colon adenocarcinoma, these cells are less tumorigenic and behave similar to normal differentiated enterocytes in vivo when cultured as confluent cells [28] . Next, we measured CTSL activity in the same panel of cell lines and observed increased CTSL activity in all malignant cancer cells tested. Again in clear contrast, only basal activity was seen in less tumorigenic and normal cell lines ( Fig. 1b ). The specificity of the CTSL assay was confirmed with inclusion of Z-FY-CHO, a specific inhibitor of CTSL [11] . These results support the utility of targeting HDAC and CTSL activities as a selective modality. 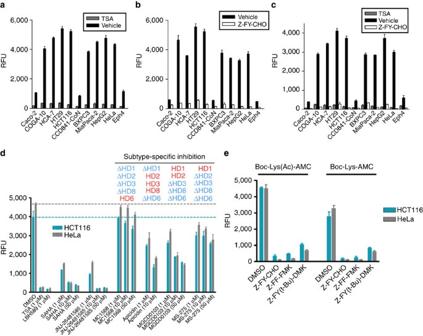Figure 1: HDAC and CTSL activities are increased in cancer cells. (a) Comparative HDAC activity of the panel of cancer and normal cell lines measured by a standard HDAC assay using substrate Boc-Lys(Ac)-AMC, either with vehicle control DMSO or HDACi TSA (1 μM). (b) Comparative live-cell CTSL activity of the same cell lines as inausing substrate Boc-Lys-AMC, either with vehicle control DMSO or CTSL inhibitor Z-FY-CHO (100 μM). (c) Comparative live-cell enzymatic activity of the same cell lines as inausing substrate Boc-Lys(Ac)-AMC, either with vehicle control DMSO, TSA (1 μM) or Z-FY-CHO (100 μM). (d) Effect of HDACi on live-cell enzymatic activity of cancer cells (HCT116 and HeLa) was examined using class I (HDAC1, 2, 3 and 8)- and class IIb (HDAC6 and 10)-specific substrate Boc-Lys(Ac)-AMC either with vehicle control DMSO or indicated HDACi. HDACi used were pan-HDACi (TSA, LBH589, SAHA and JNJ-26481585), class II-specific HDACi (MC1568) and class I HDAC subtype-specific HDACi (Apicidin, MGCD0103 and MS-275). The specificity of the subtype inhibitors is shown above the respective panels. HD, HDAC; Δ, inactive or less active (IC50>1 μM range)31. The assays were performed as inc. (e) Effect of selective CTSL inhibitors on the live-cell enzymatic activity of cancer cells (HCT116 and HeLa) was examined using substrate Boc-Lys(Ac)-AMC or Boc-Lys-AMC, either with vehicle control DMSO, Z-FY-CHO (100 μM), Z-FF-FMK (100 μM, Cathepsin L Inhibitor I, Calbiochem) or Z-FY(t-Bu)-DMK (10 μM, Cathepsin L Inhibitor III, Calbiochem). The assays were performed as inb,c. Data represent mean values of triplicate measurements±s.d. RFU, relative fluorescent units. Figure 1: HDAC and CTSL activities are increased in cancer cells. ( a ) Comparative HDAC activity of the panel of cancer and normal cell lines measured by a standard HDAC assay using substrate Boc-Lys(Ac)-AMC, either with vehicle control DMSO or HDACi TSA (1 μM). ( b ) Comparative live-cell CTSL activity of the same cell lines as in a using substrate Boc-Lys-AMC, either with vehicle control DMSO or CTSL inhibitor Z-FY-CHO (100 μM). ( c ) Comparative live-cell enzymatic activity of the same cell lines as in a using substrate Boc-Lys(Ac)-AMC, either with vehicle control DMSO, TSA (1 μM) or Z-FY-CHO (100 μM). ( d ) Effect of HDACi on live-cell enzymatic activity of cancer cells (HCT116 and HeLa) was examined using class I (HDAC1, 2, 3 and 8)- and class IIb (HDAC6 and 10)-specific substrate Boc-Lys(Ac)-AMC either with vehicle control DMSO or indicated HDACi. HDACi used were pan-HDACi (TSA, LBH589, SAHA and JNJ-26481585), class II-specific HDACi (MC1568) and class I HDAC subtype-specific HDACi (Apicidin, MGCD0103 and MS-275). The specificity of the subtype inhibitors is shown above the respective panels. HD, HDAC; Δ, inactive or less active (IC 50 >1 μM range) [31] . The assays were performed as in c . ( e ) Effect of selective CTSL inhibitors on the live-cell enzymatic activity of cancer cells (HCT116 and HeLa) was examined using substrate Boc-Lys(Ac)-AMC or Boc-Lys-AMC, either with vehicle control DMSO, Z-FY-CHO (100 μM), Z-FF-FMK (100 μM, Cathepsin L Inhibitor I, Calbiochem) or Z-FY(t-Bu)-DMK (10 μM, Cathepsin L Inhibitor III, Calbiochem). The assays were performed as in b , c . Data represent mean values of triplicate measurements±s.d. RFU, relative fluorescent units. Full size image Design and synthesis of an agent targeting HDAC and CTSL Typical fluorogenic substrates for class I HDACs consist of an ε-acetylated lysine residue (alone or in a short peptide) coupled through a carboxy-terminal amide to a fluorescent moiety such as 7-amino-4-methylcoumarin (AMC), for example, cell-permeable Boc-Lys(Ac)-AMC [29] , [30] . These synthetic substrates undergo a two-step conversion. First, HDAC deacetylates the ε-acetyl on the lysine. Second, proteases cleave the Lys-AMC amide bond to release the AMC, which fluoresces. In tissue culture-based assays, the second step is performed after cell lysis by addition of excessive amount of trypsin, which only recognizes deacetylated lysine [29] , [30] . As the deacetylated Boc-Lys-AMC was the identical substrate used in our CTSL assay, we postulated that the substrate Boc-Lys(Ac)-AMC could also be processed in live cells through the two-step conversion by endogenous HDAC and CTSL activities. To confirm whether the conversion proceeds efficiently in live cells, we monitored the levels of released AMC using Boc-Lys(Ac)-AMC without cell lysis and trypsin treatment ( Fig. 1c ). Consistent with the elevated levels of HDAC and CTSL activities, increased levels of AMC were detected in all malignant cell lines tested. Importantly, the observed effects were specifically inhibited either in the presence of TSA or Z-FY-CHO, confirming that both HDAC and CTSL activities are required for the release of AMC in live cells ( Fig. 1c ). This HDAC and CTSL dependency was further confirmed by other pan-HDACi (LBH589, SAHA and JNJ-26481585) [31] , [32] ( Fig. 1d ) and selective CTSL inhibitors (Z-FF-FMK and Z-FY(t-Bu)-DMK; Fig. 1e ). In addition, the effects of subtype-specific HDACi (Apicidin for HDAC2, 3 and 8, MGCD0103 for HDAC1 and 2, MS-275 for HDAC1, and MC1568 for class II) [31] , [33] were examined to determine as to which HDAC subtype is responsible for processing the substrate Boc-Lys(Ac)-AMC ( Fig. 1d ). Although class II HDACi MC1568 had essentially no inhibitory effect, all other class I HDACi caused partial inhibition. The results suggest that it is most likely to be the individual class I HDAC1, 2 and 3, but not Class IIb HDAC6, that are active against the substrate. Furthermore, the data indicate the possibility that class I HDACs might have additive effects against the substrate Boc-Lys(Ac)-AMC. Taken together, the data clearly indicate that the substrate Boc-Lys(Ac)-AMC can be selectively processed in live cells in a HDAC- and CTSL-dependent manner, further supporting our approach. Having established the utility of the substrate Boc-Lys(Ac)-AMC in live cells, we designed a potential compound by conjugating the substrate moiety Boc-Lys(Ac), which serves as a masking group with a cytotoxic drug ( Fig. 2a ). As a cytotoxic drug, we selected an antibiotic puromycin (Puro), a potent protein synthesis inhibitor that causes premature termination of growing polypeptide chains on ribosome [34] , and thus can rapidly kill most cells. Resistance to Puro is conferred by the Puro N-acetyl-transferase gene, pac , which is widely used as a selection marker for gene transfer [34] . Given that the cytotoxicity of Puro requires its free amino group and can be completely inactivated by the acetylation of the amino group by the pac gene product, we reasoned that this antibiotic would be an ideal candidate for the evaluation of HDAC- and CTSL-dependent drug activation. Thus, we synthesized Boc-Lys(Ac)-Puro ( Boc-KAc-Puro ) by conjugating Boc-Lys(Ac)-OH to the amino group of Puro ( Fig. 2b and Supplementary Fig. S1a,b ). 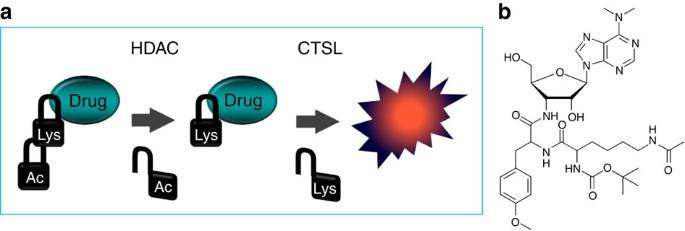Figure 2: Development of a selective anticancer agent targeting HDAC and CTSL. (a) A scheme of the selective two-step drug activation in cancer cells by HDAC and CTSL. (b) Structure of Boc-Lys(Ac)-Puro. Figure 2: Development of a selective anticancer agent targeting HDAC and CTSL. ( a ) A scheme of the selective two-step drug activation in cancer cells by HDAC and CTSL. ( b ) Structure of Boc-Lys(Ac)-Puro. Full size image In vitro activity and selectivity of Boc-KAc-Puro Next, we characterized the anticancer properties of Boc-KAc-Puro in the panel of colon cell lines. The agent impaired the proliferation of all four malignant cells, which exhibit high HDAC and CTSL activities, whereas non-malignant Caco-2 cells proliferated to confluency ( Fig. 3a ). This noteworthy feature distinguishes Boc-KAc-Puro from the general cytostatic effects seen on normal cells with most antimetabolite cancer drugs and HDACi [5] . Consistent with the effect on cell proliferation, we detected massive cell death only in the malignant cells as judged by trypan blue exclusion ( Fig. 3b ), morphological changes under phase contrast and propidium iodide (PI) staining ( Fig. 3c and Supplementary Fig. S2 ). These results indicate that the antiproliferative and cytotoxic effects of Boc-KAc-Puro are selective for malignant cells and are exclusively associated with increased levels of HDAC and CTSL activities. 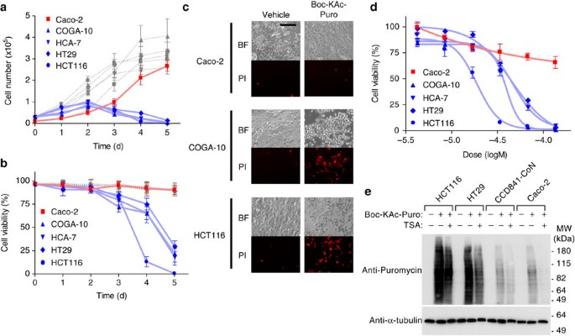Figure 3: Anticancer properties of Boc-Lys(Ac)-Puro in colon cancer cell lines. (a) The colon cancer cell lines were grown for 5 days either with vehicle control DMSO (gray symbols) or 54 μMBoc-KAc-Puro(red and blue symbols), and cell number was determined at the indicated time points. (b) The cell lines were grown as ina; cell viability was determined by trypan blue exclusion at the indicated time points and is presented as the percentage of live cells treated with vehicle control (gray symbols) orBoc-KAc-Puro(red and blue symbols). (c) The cell lines were grown as ina, and dead cells were determined after 80 h by PI signal under fluorescent microscopy. BF, bright field; PI, fluorescent PI channel; Scale bar, 50 μm (in all images). (d) Inhibition of cell viability byBoc-KAc-Purois presented in a dose–response curve format for the same cell lines as ina. The cell lines were treated with DMSO or the indicated doses of agent (4.22, 8.44, 16.9, 33.8, 67.5 or 135 μM) for 5 days followed by MTS assay. Data ina,b,drepresent mean values of triplicate measurements±s.d. (e) Levels of Puro-incorporated proteins in the cells were monitored by immunoblotting. Indicated cell lines were treated either with vehicle control DMSO orBoc-KAc-Puro(16.9 μM) in the presence or absence of TSA (0.5 μM) for 20 h, followed by preparation of cell lysates. The lower panel (anti-α-tubulin) serves as a loading control. Figure 3: Anticancer properties of Boc-Lys(Ac)-Puro in colon cancer cell lines. ( a ) The colon cancer cell lines were grown for 5 days either with vehicle control DMSO (gray symbols) or 54 μM Boc-KAc-Puro (red and blue symbols), and cell number was determined at the indicated time points. ( b ) The cell lines were grown as in a ; cell viability was determined by trypan blue exclusion at the indicated time points and is presented as the percentage of live cells treated with vehicle control (gray symbols) or Boc-KAc-Puro (red and blue symbols). ( c ) The cell lines were grown as in a , and dead cells were determined after 80 h by PI signal under fluorescent microscopy. BF, bright field; PI, fluorescent PI channel; Scale bar, 50 μm (in all images). ( d ) Inhibition of cell viability by Boc-KAc-Puro is presented in a dose–response curve format for the same cell lines as in a . The cell lines were treated with DMSO or the indicated doses of agent (4.22, 8.44, 16.9, 33.8, 67.5 or 135 μM) for 5 days followed by MTS assay. Data in a , b , d represent mean values of triplicate measurements±s.d. ( e ) Levels of Puro-incorporated proteins in the cells were monitored by immunoblotting. Indicated cell lines were treated either with vehicle control DMSO or Boc-KAc-Puro (16.9 μM) in the presence or absence of TSA (0.5 μM) for 20 h, followed by preparation of cell lysates. The lower panel (anti-α-tubulin) serves as a loading control. Full size image To further evaluate the anticancer efficacy of Boc-KAc-Puro in vitro , we performed cell viability assays ( Fig. 3d ). The dose–response curves obtained from the panel of colon cell lines indicate comparable IC 50 values (10 1 μM range) for the malignant cell lines that have high HDAC and CTSL activities ( Table 1 ). In striking contrast, the IC 50 values for non-malignant Caco-2 cells were not measurable, as sufficient inhibition of cell viability was not achieved with doses up to 135 μM, which is >30 times higher than the dose of the parental drug Puro effective in these cells ( Supplementary Fig. S3 ). Other normal cell lines with low HDAC and CTSL activities (CCD841-CoN and Eph4) showed similar pattern of dose–response to Caco-2 ( Supplementary Fig. S4 ), proving that the observed inactivity of the agent is not limited to Caco-2. Furthermore, Boc-KAc-Puro was able to kill other malignant cell lines, including pancreatic, liver and cervical cancers ( Table 1 and Supplementary Fig. S5 ), consistent with their increased HDAC and CTSL activities ( Fig. 1a–c ). These results suggest that the agent could be used as an effective regimen for a broad spectrum of cancers. Taken together, our results demonstrate that Boc-KAc-Puro exhibits a high degree of selectivity towards cells expressing increased HDAC and CTSL activities, which is a characteristic of malignant cancer over non-malignant and normal cells with basal HDAC and CTSL activities. Table 1 IC 50 values for Boc-KAc-Puro. Full size table We examined the mechanism of cell death induced by Boc-KAc-Puro . As a Tyr-tRNA mimetic, Puro enters the ribosome A site and blocks peptide chain elongation by covalent incorporation into the C terminus of nascent polypeptide chains [35] . In contrast, the prodrug is unable to do so, as its active centre amino group is masked. This allows us to monitor active Puro conversion in cells by immunological detection of Puro-labelled proteins using anti-Puro antibody [36] . To confirm that Boc-KAc-Puro is selectively converted into Puro in malignant cancer cells resulting in their death, we assessed the level of Puro incorporation by immunoblotting using cell lysates from cells treated with the agent. The intensity of Puro incorporation was substantially greater in malignant cancer cells (HCT116 and HT29) compared with normal and non-malignant cells (CCD841-CoN and Caco-2; Fig. 3e ) in accordance with their sensitivity to the agent. The compromised intensity in the presence of TSA was at least partially attributable to the specific requirement of HDAC activity for the prodrug activation. When these cells were treated with parental Puro, there was no difference in terms of Puro incorporation regardless of TSA treatment ( Supplementary Fig. S6 ). This is consistent with the ability of parental Puro to kill all of these cells examined. The results indicate that the agent can be selectively converted into Puro in malignant cancer cells, leading to their death by a Puro-dependent mode of action. In vivo tumour xenograft growth inhibition To assess in vivo anticancer efficacy of the agent, we used mouse xenograft models bearing human colon cancer cell lines (HCT116 and HT29). First, HCT116 cells were subcutaneously injected into the lower flank of mice, then dosing was initiated when small palpable tumours had developed (>3 mm in diameter). Boc-KAc-Puro was daily administered intraperitoneally at 50 and 150 mg kg −1 per dose for 10 days. The agent caused a dose-dependent inhibition of tumour growth ( Fig. 4a ). In this model, animals treated with the prodrug developed significantly smaller tumour mass in comparison with the animals treated with acidified saline control ( P <0.001; two-tailed Student’s t test). Furthermore, daily intraperitoneal administration of the prodrug as high as 150 mg kg −1 per dose for 10 days appeared well tolerated as judged by weight loss determination ( Fig. 4b ). Similar results were obtained using HT29 cells at 150 mg kg −1 per dose ( Fig. 4c,d ). These results clearly demonstrate in vivo anticancer efficacy of the prodrug Boc-KAc-Puro without severe off-target systemic toxicity. 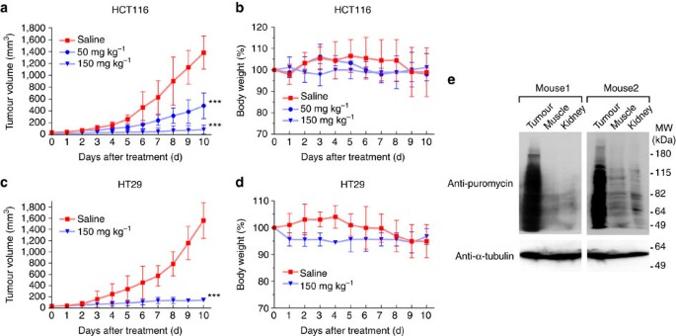Figure 4:In vivoanticancer efficacy of Boc-KAc-Puro. (a) Tumour growth in HCT116 xenograft model. Animals were treated with acidified saline control orBoc-KAc-Puro(50 or 150 mg kg−1). Values are mean±s.d. (n=5 mice per group). ***P<0.001 compared with the control group.P=0.000716 (50 mg kg−1),P=0.000349 (150 mg kg−1) at 10 days (two-tailed Student’st-test). (b) Body weight change during the treatment inawas monitored as a sign of general animal health. Values are mean±s.d. (c) Tumour growth in HT29 xenograft model. Animals were treated with acidified saline control orBoc-KAc-Puro(150 mg kg−1). Values are mean±s.d. (n=5 mice per group). ***P<0.001 compared with the control group.P=0.000514 (150 mg kg−1) at 10 days (two-tailed Student’st-test). (d) Body weight change during the treatment incwas monitored as a sign of general animal health. Values are mean±s.d. (e) Levels of Puro-incorporated proteins were monitored by immunoblotting. Animals bearing HT29 xenograft tumour were given daily intraperitoneal administration of the prodrug at 150 mg kg−1per dose for 3 days, followed by preparation of tissue lysates. The lower panel (anti-α-tubulin) served as a loading control. Figure 4: In vivo anticancer efficacy of Boc-KAc-Puro. ( a ) Tumour growth in HCT116 xenograft model. Animals were treated with acidified saline control or Boc-KAc-Puro (50 or 150 mg kg −1 ). Values are mean±s.d. ( n =5 mice per group). *** P <0.001 compared with the control group. P =0.000716 (50 mg kg −1 ), P =0.000349 (150 mg kg −1 ) at 10 days (two-tailed Student’s t -test). ( b ) Body weight change during the treatment in a was monitored as a sign of general animal health. Values are mean±s.d. ( c ) Tumour growth in HT29 xenograft model. Animals were treated with acidified saline control or Boc-KAc-Puro (150 mg kg −1 ). Values are mean±s.d. ( n =5 mice per group). *** P <0.001 compared with the control group. P =0.000514 (150 mg kg −1 ) at 10 days (two-tailed Student’s t -test). ( d ) Body weight change during the treatment in c was monitored as a sign of general animal health. Values are mean±s.d. ( e ) Levels of Puro-incorporated proteins were monitored by immunoblotting. Animals bearing HT29 xenograft tumour were given daily intraperitoneal administration of the prodrug at 150 mg kg −1 per dose for 3 days, followed by preparation of tissue lysates. The lower panel (anti-α-tubulin) served as a loading control. Full size image To assess whether the prodrug is selectively activated at tumour sites in vivo , we monitored levels of Puro incorporation into polypeptides in tumours and normal tissues, including the muscle underneath the tumours and the kidney, one of the major excretion sites for drug metabolites. Animals bearing HT29 xenograft tumour were given daily intraperitoneal administration of the prodrug at 150 mg kg −1 per dose for 3 days followed by preparation of tissue lysates for immunological detection of Puro-labelled proteins. The intensity of Puro incorporation was substantially greater in tumours compared with that in normal muscle, kidney ( Fig. 4e ) and intestine ( Supplementary Fig. S7 ), further supporting tumour-specific activation of the agent in vivo . The results indicate that the agent can be selectively converted into Puro in tumour tissues, leading to their growth inhibition by Puro-dependent mode of action. In this report, we describe the design, synthesis and characterization of Boc-KAc-Puro , a novel prodrug targeting increased HDAC and CTSL activities in malignant tumours. Anticancer efficacy of the agent is evidenced by its ability to inhibit tumour growth in vivo without severe adverse effects. Notably, this approach is potentially advantageous, because the simple small-molecule masking group could be readily applied to many other cytotoxic agents, including chemotherapeutic drugs currently used in the clinic. For example, amide coupling-based prodrugs of gemcitabine and cytarabine were developed by masking their amino group [37] , [38] . Thus, introduction of the Boc-Lys(Ac) group to their amino group should be technically feasible for evaluation of their improved efficacy. In addition, when coupled with imaging probes, the masking group could be viable tools for bioimaging and non-invasive diagnosis of cancer cells. Imaging probes, including Puro-based radiopharmaceuticals [39] and fluorescent agents [40] , could be modified to highly specific and safe probes for detection of cancer cells in the body. One might wonder how the fluorogenic substrate Boc-Lys(Ac)-AMC and the prodrug can be serially activated by the spatially separated enzymes HDAC and CTSL in the intact cells. Boc-Lys(Ac)-AMC and the deacetylated product Boc-Lys-AMC were shown to be cell permeable and freely diffusible inside the intact cells [30] . Similarly, Puro and the prodrug are water-soluble small molecules (as hydrochloride salt) that are also cell permeable and can diffuse rapidly through the aqueous cytosol in the cell. Thus, it is possible that the serial activation process by the two enzymes takes place in different subcellular locations through simple passive diffusion, regardless of the nucleus or the cytoplasm. The significant effect on tumour growth inhibition in vivo with minimal toxicity by the agent supports our strategy as a monotherapy. Further optimizations, including drug formulation, administration route, dose, frequency and exposure duration, as well as detailed pharmacokinetics, pharmacodynamics, toxicology and drug resistance studies, are warranted to maximize the full potential of the agent for clinical settings. Our observation that malignant cancer cells exhibit high levels of HDAC and CTSL activities has important implications for the potential use of their combined enzymatic activities as a selective modality for delivering therapeutics to their targets. By utilizing a small-molecule masking group, we were able to materialize a prototypic agent specifically activated by these enzymes in cancer cells. In conclusion, our work raises the possibility that targeting elevated HDAC and CTSL activities in malignant cancer cells will serve as a promising strategy for anticancer drug development. Cell culture Colon cancer (Caco-2, COGA-10, HCA-7, HT29 and HCT116), normal colon CCD841-CoN, pancreatic cancer (MiaPaca-2 and BXPC3), liver cancer HepG2, and cervical cancer HeLa and normal mouse mammary epithelial Eph4 cell lines were maintained in Iscove’s modified Dulbecco’s medium (Invitrogen) supplemented with 10% fetal bovine serum and 100 U ml −1 penicillin/streptomycin at 37 °C with 5% CO 2 atmosphere. Enzymatic assays Tissue culture-based standard HDAC assays were performed by commercially available fluorimetric HDAC assay kit (SensoLyte, AnaSpec) according to the manufacturer’s instruction, with modification of using 25 μM Boc-Lys(Ac)-AMC (Bachem) as a substrate and measuring parameter (Ex/Em=355 nm/460 nm) for AMC. Basically, HDAC substrate 25 μM Boc-Lys(Ac)-AMC (either with dimethyl sulphoxide (DMSO) or 1 μM TSA (Sigma)) was applied to the overnight culture seeded from 6 × 10 4 cells in 100 μl medium in 96-well tissue culture plates, followed by 2–3 h incubation at 37 °C with 5% CO 2 atmosphere. Next, the deacetylation reaction was terminated by addition of HDAC developer solution containing cell lysis buffer and trypsin reagents. After 15 min incubation at room temperature, the fluorescent signal of AMC was measured by SpectraMax M5 microplate reader (Molecular Devices) at Ex/Em=355 nm/460 nm. Live-cell lysyl endopeptidase assay was performed by applying the substrate 25 μM Boc-Lys-AMC (Bachem; either with DMSO or 100 μM Z-FY-CHO (Cathepsin L Inhibitor II, Calbiochem)) to the overnight culture seeded from 6 × 10 4 cells in 100 μl medium in 96-well tissue culture plates, followed by 20 h incubation at 37 °C with 5% CO 2 atmosphere, then the fluorescent signal of AMC was measured. Live-cell enzymatic assay using Boc-Lys(Ac)-AMC was performed by applying the substrate 25 μM Boc-Lys(Ac)-AMC (either with DMSO, 1 μM TSA or 100 μM Z-FY-CHO) to the overnight culture seeded from 6 × 10 4 cells in 100 μl medium in 96-well tissue culture plates, followed by 20 h incubation at 37 °C with 5% CO 2 atmosphere, then the fluorescent signal of AMC was measured. Experiments were repeated at least three times. HDAC inhibitors Apcidin and SAHA were purchased from Cayman Chemical. LBH589, JNJ-26481585, MGCD0103, MS-275 and MC1568 were purchased from Selleck USA. Cell viability assays Cell number was determined by cell counting using improved Neubauer haemocytometer. Cell viability was calculated as the number of viable cells divided by the total number of cells using Trypan Blue Stain (Invitrogen) to distinguish non-viable cells. Data were obtained from duplicated samples with quadruplicate measurements. MTS (3-(4,5-dimethylthiazol-2-yl)-5-(3-carboxymethoxyphenyl)-2-(4-sulphophenyl)-2H-tetrazolium))-based cell viability assay was performed using CellTiter 96 AQueous Cell Proliferation Assay (Promega) according to the manufacturer’s instruction. Either 1 μl of DMSO alone or variable concentrations of Boc-KAc-Puro or Puro (TOKU-E) in DMSO were added to the cell lines seeded at 5 × 10 4 cells per well in 96-well tissue culture plates in 100 μl of the growth medium, followed by 3–5 days incubation at 37 °C with 5% CO 2 atmosphere. Next, 20 μl of the MTS reagent was added to each well. After additional 2–3 h incubation, the absorbance of the formazan at 490 nm was measured by the microplate reader. Per cent cell viability was expressed relative to the wells containing cells treated with DMSO alone. Data were obtained from triplicate measurements. The IC 50 values (the concentration resulting in 50% inhibition) of Boc-KAc-Puro were determined by dose–response curve analysis (GraphPad Prism software). Experiments were repeated at least three times. Determination of non-viable cells using PI staining was performed by adding 1 μg ml −1 of PI solution (Sigma) to the cell culture before the examination under fluorescence microscopy (Axiovert 3, Carl Zeiss) through a × 32 objective equipped with a digital imaging processor (Infinity 3, Lumenera). Immunological detection of Puro-labelled proteins Cultured cells or tissue samples were sonicated in RIPA lysis buffer (1% NP-40, 0.1% SDS, 50 mM Tris–HCl, pH 7.4, 150 mM NaCl, 0.5% sodium deoxycholate, 1 mM EDTA) supplemented with phenylmethylsulphonyl fluoride and protease inhibitor cocktail (Roche) on ice, followed by clarification. Protein lysates were separated on SDS polyacrylamide gels and transferred onto nitrocellulose membranes (Whatman). The primary antibodies used were anti-Puro (1:5,000 dilution, 3RH11, KeraFAST) and anti-α-tubulin (1:4,000 dilution, Sigma-Aldrich). Proteins of interest were detected with anti-mouse secondary antibody by chemiluminescence (ECL Kit, GE Healthcare Life Sciences). Original full-blot images were provided for the partially cropped blots ( Supplementary Fig. S8 ). In vivo studies All in vivo experiments were conducted in accordance with the guidelines and protocol approved by the Institutional Animal Care and Use Committee of Stony Brook University. Athymic mice (NCr, female, age 6 weeks, Taconic) were subcutaneously injected with 5 × 10 5 cells (HCT116 or HT29) into the lower flank, then treatment was initiated when small palpable tumours had developed (>3 mm in diameter). Either Boc-KAc-Puro in 150 mM HCl (pH 2 adjusted by NaOH) or acidified saline (pH 2) as control was daily administered intraperitoneally for 10 days. Tumour volumes and body weight were monitored daily. Tumour volume was estimated by the equation vol=( a × b 2 )/2, where vol, a and b represent volume (mm 3 ), the length of the major axis (mm) and the length of the minor axis (mm), respectively. Data were expressed as mean±s.d. Synthesis of Boc-KAc-Puro Materials: α-Boc-Lys(ε-Ac)-OH and Puro dihydrochloride were purchased from Bachem and TOKU-E, respectively. 1-ethyl-3-(3-dimethylaminopropyl) carbodiimide hydrochloride (EDC·HCl) and 1- hydroxybenzotriazole (HOBt·H 2 O) were purchased from Advanced Chem Tech. Dichloromethane (DCM) and dimethylformamide (DMF) were obtained from EMD Chemical. DMF was dried and purified by solvent pushstill (SG water USA LLC, Nashua, NH). 1 H NMR data are reported as chemical shift in p.p.m. (multiplicity, coupling constant in Hz, integration and tentative assignment). 13 C NMR data are reported as chemical shift in p.p.m. (tentative assignment). Assignments are based on expected chemical shifts, multiplicities and coupling constants. Method: A mixture of Puro dihydrochloride (50 mg, 0.092 mmol), α-Boc-Lys(ε-Ac)-OH (31 mg, 0.11 mmol), EDC·HCl (21 mg, 0.11 mmol), HOBt·H 2 O (17 mg, 0.11 mmol) and DIEA (N,N-diisopropylethylamine; 18 μl, 0.11 mmol) was stirred in DMF (10 ml) at room temperature for 18 h. After concentrating the solution under reduced pressure, the residue was dissolved in DCM. The DCM solution was washed with H 2 O three times, dried over Na 2 SO 4 and concentrated. The crude oil was purified by silica-gel column chromatography using a linear gradient from 5 to 10% MeOH in DCM and dried to yield α-Boc-Lys(ε-Ac)-Puro as a white solid (55 mg, 75% yield): mp: 182–183 °C; 1 H NMR (500 MHz, DMSO) δ 8.43 (s, 1H, H-29), 8.22 (s, 1H, H-32), 8.15 (d, J =7.7 Hz, 1H, H-8′), 7.74 (d, J =7.1 Hz, 2H, H-2′, H-23′), 7.15 (d, J =8.4 Hz, 2H, H-17), 6.86 (d, J =8.3 Hz, 1H, H-9′), 6.80 (d, J =8.6 Hz, 2H, H-16, H-20), 6.03 (d, J =4.6 Hz, 1H, H-28), 5.98 (d, J =2.8 Hz, 1H, H-27), 5.18 (t, J =5.4 Hz, 1H, H-22), 4.60 (dd, J =13.6, 8.1 Hz, 1H, H-7), 4.52–4.39 (m, 2H, H-25, H-26), 3.98–3.76 (m, 2H, H-24), 3.70 (s, 3H, H-14), 3.69 –3.40 (m, 6H, H-34, H-35), 3.02–2.86 (m, 3H, H-3, H-21), 2.76 (dd, J =13.7, 8.7 Hz, 1H, H-21), 1.77 (s, 3H, H-1), 1.52–1.38 (m, 2H, H-6), 1.38–1.32 (s, 9H, H-11, H-12, H-13), 1.33–1.05 (m, 4H, H-4, H-5) p.p.m. 13 C NMR (101 MHz, DMSO) δ 169.5 (C-8, C-23), 158.4 (C-9), 155.8 (C-2), 154.8 (C-33), 152.4 (C-32), 150.2 (C-31), 138.4 (C-29), 138.3 (C-15), 131.0 (C-17, C-19), 129.8 (C-18), 120.2 (C-30), 114.0 (C-16, C-20), 90.0 (C-28), 78.8 (C-10, C-25), 73.8 (C-27), 61.5 (C-24), 55.6 (C-26), 55.3 (C-7), 54.5 (C-22), 51.0 (C-14), 40 ((C-34, C-35, underneath DMSO peak), 39.1 (C-3), 38.2 (C-21), 32.5 (C-6), 29.5 (C-4), 28.9 (C-11, C-12, C-13), 23.7 (C-5), 23.4 (C-1); MS ( m/z ): [M] + calcd for C 35 H 51 N 9 O 9 , 742.38; found, 742.47. Spectral data are presented in Supplementary Fig. S1 . Statistical analyses For the in vivo experiments, a two-tailed Student’s t -test was used to calculate statistical significance of the observed differences. P <0.05 was considered statistically significant. How to cite this article: Ueki, N. et al. Selective cancer targeting with prodrugs activated by histone deacetylases and a tumour-associated protease. Nat. Commun. 4:2735 doi: 10.1038/ncomms3735 (2013).